Blood-clotting-inspired reversible polymer–colloid composite assembly in flow Blood clotting is a process by which a haemostatic plug is assembled at the site of injury. The formation of such a plug, which is essentially a (bio)polymer–colloid composite, is believed to be driven by shear flow in its initial phase, and contrary to our intuition, its assembly is enhanced under stronger flowing conditions. Here, inspired by blood clotting, we show that polymer–colloid composite assembly in shear flow is a universal process that can be tailored to obtain different types of aggregates including loose and dense aggregates, as well as hydrodynamically induced ‘log’-type aggregates. The process is highly controllable and reversible, depending mostly on the shear rate and the strength of the polymer–colloidbinding potential. Our results have important implications for the assembly of polymer–colloid composites, an important challenge of immense technological relevance. Furthermore, flow-driven reversible composite formation represents a new paradigm in non-equilibrium self-assembly. Polymer–colloid composites represent an attractive class of hybrid materials in which one can tailor their properties by exploiting the individual and collective properties of both components [1] , [2] , [3] , [4] . However, uniformly dispersing colloids in polymer matrices, and vice versa, has represented a challenge that requires careful tuning of the interactions and the processing conditions [5] , [6] , [7] . Nature, on the other hand, can assemble to perfection complex composite materials for a variety of functions. For example, the abalone shell is made out of calcium carbonate and organic matrices, or bone that is composed of calcium phosphate and collagen fibres, both of which display excellent mechanical properties [8] , [9] . In most cases, these materials are constructed very slowly, and are perhaps not viable for technological applications. There are some instances in nature, however, in which forming a composite very rapidly is necessary, and such conditions are met during blood clotting. During this process, our body forms a polymer–platelet composite called the plug within seconds of injury [10] , [11] . This aggregate composed of von Willebrand factor (vWF), which is a long biopolymer, and platelets forms the scaffold for the formation of a clot at the site of the lesion. Both vWF and platelets are necessary to form the plug, and a lack in activity of vWF leads to the most common hereditary disease that ~1% of the population has, the so-called von Willebrand disease [12] . Once the plug has been assembled, a fibrin chemically crosslinked network is polymerized in-situ through a large network of chemical reactions (for a more detailed description see ref. 13 ). Interestingly, the propensity for forming a thrombus is highly regulated by fluid flows, increasing as you increase the flow strength for shear rates as high as 10,000 s −1 (refs 14 , 15 ). Note that this behaviour cannot be sustained indefinitely, and for extremely high shear rates one expects flow-induced dissolution of the aggregates. The enhancement in thrombus formation is particularly true in the presence of vWF, and it has been shown that the formation of the plug can be driven purely by flow in a reversible fashion [16] , [17] , [18] . Such behaviour is completely contrary to our intuition based on the fact that we typically use strong flows to disintegrate or dissolve matter, and thus the clotting scenario in which flow controls the reversible assembly of complex composites (with presumably tailored properties) represents a completely new aggregation paradigm that cannot be understood in terms of purely diffusion-limited and/or reaction-limited aggregation concepts. In the later cases, flow just accelerates the aggregation process but the aggregates are not reversible. Inspired by the process of blood clotting, here we explore with simulations and experiments the flow-driven self-assembly of polymer–colloid composites (see Fig. 1 ). Our model system, which mimics the blood, consists of a dilute polymer and colloid mixture. The colloids can bind to the polymer through specific interactions, as is known to occur between von Wilebrand Factor and platelets in blood. We find that such polymer–colloid system exhibits reversible aggregation regulated by the shear forces, and the aggregation process is universal. 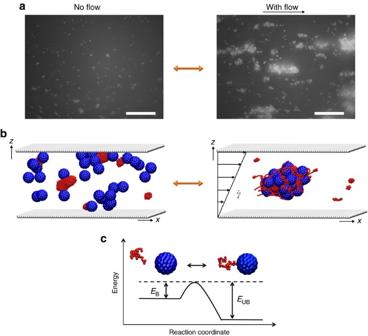Figure 1: Schematics of shear-induced aggregates and Bell interaction model. (a) Combined interference contrast microscopy and fluorescence images of vWF–colloids mixtures before (left) and after applying flow (right). At a critical shear rate of≈4,000s−1(right) reversible aggregates appear rolling on the vWF-coated surface, dissolving after reducing the shear rate (as shown inSupplementary Movie 2). Scale bars correspond to 50 μm. Number of experimental repeats=6. (b) Simulation snapshots for polymer and colloid mixtures without (left) and with shear flow (right). Red beads represent the polymers, and blue beads represent the discrete binding sites on the colloid surfaces. (c) The energy landscape for a single associating pair of one monomer and one colloid binding site. The energy to form this bond is given byEB, and the barrier to break this bond is given byEUB. Figure 1: Schematics of shear-induced aggregates and Bell interaction model. ( a ) Combined interference contrast microscopy and fluorescence images of vWF–colloids mixtures before (left) and after applying flow (right). At a critical shear rate of ≈4,000s −1 (right) reversible aggregates appear rolling on the vWF-coated surface, dissolving after reducing the shear rate (as shown in Supplementary Movie 2 ). Scale bars correspond to 50 μm. Number of experimental repeats=6. ( b ) Simulation snapshots for polymer and colloid mixtures without (left) and with shear flow (right). Red beads represent the polymers, and blue beads represent the discrete binding sites on the colloid surfaces. ( c ) The energy landscape for a single associating pair of one monomer and one colloid binding site. The energy to form this bond is given by E B , and the barrier to break this bond is given by E UB . Full size image Flow-driven self-assembly of polymer–colloid composites To study the aforementioned polymer–colloid system, we consider a mixture of homopolymers with volume fraction φ p ≈0.5% and spherical colloids with volume fraction φ c ≈3%. These volume fractions correspond to the volume fractions of vWF and platelets in blood, as was used in the experiments. Notice that under these dilute conditions without flow, the polymers and the colloids do not aggregate even if they have attractive interactions between them. The polymers are simulated by a simple bead-spring model, and the colloids are simulated as hard spheres. The last assumption deviates from the actual soft-colloid properties of platelets, but as will be shown below, such a condition is not necessary for assembly. In fact, as shown in Fig. 1a , flow-driven composite assembly also occurs if we exchange the actual platelets by functionalized hard colloids in the experiments (see Supplementary Fig. S1 for a comparison with the platelet experiments). The solvent quality for the vWF, which is believed to be in a collapse state, is taken into account by using a Lennard–Jones potential between non-adjacent monomers along the chain (see Methods ). Such a model for collapsed polymers has been shown to be a good model for vWF [16] . Under normal pH and temperature conditions, it was found that the attractive well strength of u =2.08 k B T (where k B is the Boltzmann constant and T is the temperature) in the Lennard–Jones potential compared the best against the experimental data. Hence, for collapsed vWF polymers we will use such value. For comparison purposes, we also study Θ polymers, which correspond to u =0.41 k B T [19] , [20] . The monomers interact with the colloids at discrete binding sites on the colloid surfaces that mimic the actual GPIb-α receptor on the surface of platelets that specifically binds to the A1 domain of vWF [10] , [11] , [12] . The binding process is modelled through the classical model of Bell [21] (see Fig. 1c ), which is a new method to include microscopic-associating reactions in highly coarse-grained polymer simulations [22] , [23] , [24] . In the Bell model, the formation and disassociation of bonds is controlled by the binding and unbinding energy barriers E B and E UB , as well as the tension applied on the bonds (see Methods ). For the particular case of vWF and platelets, the binding energy landscape is not so well studied, but it is believed that the association is relatively fast. Hence, we fix E B =1 k B T , which ensures fast binding dynamics for bond formation. On the other hand, we consider different values of E UB , which controls the bond strength and bond lifetime (unbinding time scale) accordingly. For simplicity, we assume the polymers to be 40 monomers long, corresponding to the typical size of a vWF active fibre, and also we only consider spherical colloids of a size corresponding to 2 μm, equivalent to the size of platelets. Finally, the system is coupled to a fluctuating Lattice Boltzmann (LB) solver on the background that is used to study the aggregation under flow, ensuring the correct dissipative and fluctuating hydrodynamics [25] , [26] . To study the effects of shear flow on the polymer and colloid aggregation, we impose simple shear flow with dimensionless shear rates ranging from τ=0.01−2, where τ is the monomer diffusion time (see Methods ). For the particular case of vWF, τ is of the order of 10 −4 s. The aggregation size is characterized by counting the average number of bonds formed between polymers and colloids. 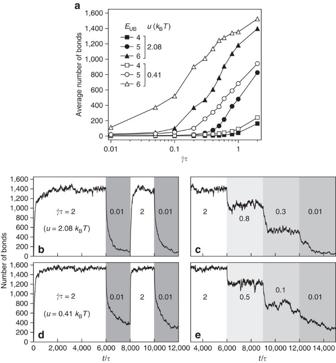Figure 2: Average aggregation sizes and reversibility tests. (a) Average number of polymer–colloid bonds as a function of the imposed shear ratesτ with different unbinding energiesEUBand types of polymers (u=2.08kBTfor collapsed polymers and 0.41kBTfor Θ polymers). (b–e) Number of polymer–colloid bonds as a function of the simulation timet/τwhen suddenly switching the shear rates between the maximum and minimum values (b,d), or gradually decreasing the shear rates (c,e). (b,c) Are for the mixtures of the collapsed polymers; (d,e) are for the Θ polymers. Figure 2a shows the average ‘aggregation size’ as a function of the shear rates for different E UB and u . In all conditions, the aggregation size increases with increasing shear rates. As mentioned earlier, this is a counterintuitive result at first sight as one would expect that stronger shear flow disassembles the aggregates more readily. Such is the case for pure colloidal aggregates in the diffusion-limited regime (see Supplementary Fig. S2 ). Nevertheless, using a simple scaling argument, we can show that rotation of the colloids in shear flow is in fact enhancing the wrapping of the polymer chains onto the colloid surfaces, which then enhances the aggregation. Note, however, that the shear-induced aggregation cannot be sustained indefinitely, and for extremely high shear rates one expects flow-induced dissolution of the aggregates (see Supplementary Fig. S3 ). The shear-induced aggregation is also observed in the experiments using vWF and platelets mixtures (see Supplementary Fig. S1 ). Platelets can be substituted with hard colloids of size ≈2 μm that are functionalized on their surface with the anti-vWF antibody that binds vWF (see Fig. 1a ). Without addition of vWF to the samples, the flow-driven composite assembly could not be detected using platelets and colloids, respectively (see Supplementary Fig. S4 ). Merely single platelets or colloids specifically interact with the vWF biofunctionalized surface. To further address the specificity of reversible vWF–platelet assembly under flow conditions, we rerun the vWF–platelet mixture experiments supplemented with a monoclonal inhibitor of GPIb-α receptor. As shown in the Supplementary Fig. S5 , no colloid–polymer composite assembly was detectable. Figure 2: Average aggregation sizes and reversibility tests. ( a ) Average number of polymer–colloid bonds as a function of the imposed shear rates τ with different unbinding energies E UB and types of polymers ( u =2.08 k B T for collapsed polymers and 0.41 k B T for Θ polymers). ( b – e ) Number of polymer–colloid bonds as a function of the simulation time t/τ when suddenly switching the shear rates between the maximum and minimum values ( b , d ), or gradually decreasing the shear rates ( c , e ). ( b , c ) Are for the mixtures of the collapsed polymers; ( d , e ) are for the Θ polymers. Full size image Comparing the effects of the unbinding energies ( E UB ), we observe that, for both collapsed and Θ polymers at a given shear rate, the higher the E UB , the larger the aggregates. This result is expected as for higher unbinding energies it is harder to break the polymer and colloid bonds, and easier for the aggregates to grow. Comparing the effects of the solvent properties ( u ), we observe that mixtures containing Θ polymers ( u =0.41 k B T ) form larger aggregates at a smaller shear rate compared with mixtures using collapsed polymers ( u =2.08 k B T ). This phenomenon is owing to the fact that collapsed polymers form compact globules at low shear rates. Thus, most of the monomers are hidden within the interior and the probability for the interactions between the monomers and the colloid-binding sites decreases substantially. One of the interesting features of these polymer–colloid composites is that the shear-induced aggregation is reversible. That is, the shear-induced aggregation disappears when the imposed shear flow is removed. Figure 2b–e shows the results of different reversibility tests for the mixtures of both the collapsed ( Fig. 2b ) and the Θ polymers ( Fig. 2d ). In these plots, we show the aggregation sizes (number of polymer and colloid bonds) as a function of the simulation time t/τ , where we either rapidly switch the shear rates between the maximum and minimum values ( Fig. 2b ), or gradually decrease the shear rates ( Fig. 2c and e ). In both tests, the reversibility of the shear-induced aggregation is clearly observed. The reversibility of this shear-induced polymer and colloid aggregation was also observed in the experiments ( Supplementary Movies 1 and 2 ). Structures of the polymer–colloid aggregates The properties of the shear-induced aggregates can be tailored by the strength of the flow. For example, by careful inspection of the radial distribution function g(r) (where r is the distance between the centre of mass of the colloids), as well as by visual inspection, we find four distinct microstructures ( Fig. 3 ). These structures are observed for both mixtures of the collapsed and Θ polymers. At low shear rates, there is no obvious aggregation ( Fig. 3a ). For low to intermediate shear rates ( τ≈0.2−0.5 in the case of bad solvent, and τ≈0.05−0.1 for the Θ polymers), the polymers and colloids start to form loose aggregates ( Fig. 3b and f ), as can be seen from the visualizations and the increasing peaks in the g(r) plots at r /2 r c <2, where r c is the radius of the colloids. Increasing the shear rates further ( τ≈0.6−1 for collapsed polymers and τ≈0.2−0.8 for Θ polymers), the aggregates transfer from the loose structures to a more compact morphology ( Fig. 3c ), as can be seen by visual inspection. In addition, in the g(r) plots for the compact aggregates, the relative colloid distribution is highly concentrated within r /2 r c <3. For the highest shear rates ( τ>2 for collapsed polymers and τ>1 for Θ polymers), we find that the aggregates form parallel strings perpendicular to the flow direction ( Fig. 3d ). This special alignment of the colloids is caused by the strong hydrodynamic coupling between the colloids, an effect that has been very recently observed in pure colloidal systems under strong shear flows [27] and also in blood as shown in Supplementary Movies 1 and 2 . 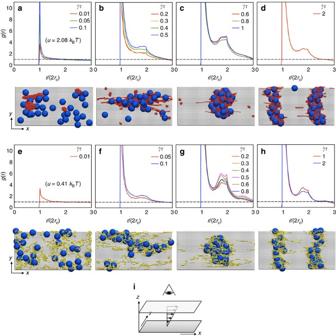Figure 3: Microstructures of shear-induced aggregates. The radial distribution functionand characteristic snapshots corresponding to the different aggregate types. (a–d) are for the mixtures containing collapsed polymers; (e–h) are for the Θ polymers. The four distinct microstructures are: (1) no aggregates (a,e), (2) loose aggregates (b,f), (3) compact aggregates (c,g) and (4) ‘log’ aggregates (d,h). (i) Sketch of the observation viewpoint for the snapshots. Figure 3: Microstructures of shear-induced aggregates. The radial distribution function and characteristic snapshots corresponding to the different aggregate types. ( a – d ) are for the mixtures containing collapsed polymers; ( e – h ) are for the Θ polymers. The four distinct microstructures are: (1) no aggregates ( a , e ), (2) loose aggregates ( b , f ), (3) compact aggregates ( c , g ) and (4) ‘log’ aggregates ( d , h ). ( i ) Sketch of the observation viewpoint for the snapshots. Full size image Universal assembly behaviour in shear flow Finally, by using a simple scaling argument to describe how the shear flow can enhance the polymer and colloid aggregation, we can show that this phenomenon is universal. In this particular problem, the most relevant time scales are: (1) the time scale associated with rotation and collision of the colloids τ 1 ≈1/ that is inversely proportional to the applied shear rate , and (2) the unbinding time scale for the polymer–colloid bonds τ 2 ≈ τ 0 exp( E UB / k B T ), where τ 0 is a resting time between consecutive binding and unbinding attempts. Notice that τ 2 increases exponentially with E UB . If τ 2 > τ 1 , then we expect aggregation as bonded polymers will effectively render the colloids as sticky colloids. Thus, if we plot the data in terms of τ 2 / τ 1 , instead of just the shear rate (as in Fig. 2a ), we expect to see the formation of the aggregates to collapse into a single master curve. This is clearly the case as is shown in Fig. 4a , where we plot the average aggregation size (number of bonds) as a function of τ 2 / τ 1 for collapsed polymers ( u =2.08 k B T ). All the data collapses nicely onto a universal curve, and the aggregation sizes start to grow when τ 2 / τ 1 >~1. For the Θ polymers ( u =0.41 k B T ), it is possible that the initial polymer and colloid interaction includes more than one bond (as the chains form random coils) introducing a cooperative factor n b ( Fig. 4b insert). In this particular case, we find that the instantaneous number of polymer–colloid bonds is on average ~2. This can be seen clearly when we collapse the data by introducing a correction term for this cooperative factor in the unbinding time scale such that τ 2 ≈ τ 0 exp( n b E UB / k B T ) where n b is the number of bonds to break at the same time in order to detach the polymer. Using n b =2, a universal curve is obtained for the average aggregation sizes as a function of τ 2 / τ 1 for the mixtures of the Θ polymers and colloids ( Fig. 4b ). 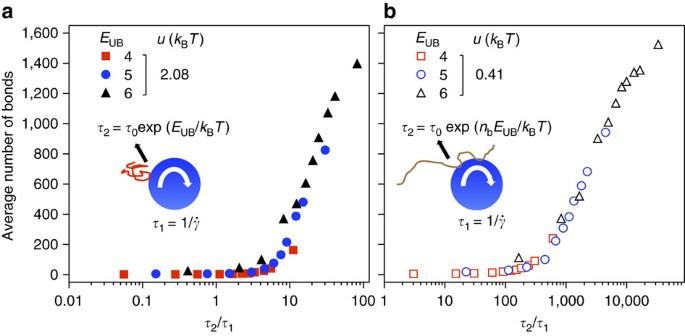Figure 4: Universal scaling for aggregation sizes. Average number of polymer–colloid bonds as a function of the ratio of the unbinding time scaleτ2≈τ0exp(nbEB/kBT) and the rotation time scale τ1≈1/. In (a) the cooperative factornb=1 for collapsed polymers, and in (b) the cooperative factornb=2 for Θ polymers. (Insets ina,b: schematics of the physical pictures for constructing the scaling relations.) Figure 4: Universal scaling for aggregation sizes. Average number of polymer–colloid bonds as a function of the ratio of the unbinding time scale τ 2 ≈ τ 0 exp( n b E B / k B T ) and the rotation time scale τ 1 ≈1/ . In ( a ) the cooperative factor n b =1 for collapsed polymers, and in ( b ) the cooperative factor n b =2 for Θ polymers. (Insets in a , b : schematics of the physical pictures for constructing the scaling relations.) Full size image The physical picture behind our scaling argument is based on understanding what are the necessary conditions for composite formation. In order to start the formation of an aggregate, a polymer must link two (or more) colloids. The first step is then for a polymer to form one (or more) bond(s) with a single colloid. Note that each of the repeating units (or ‘monomers’) in vWF can only form one bond with the platelets through the vWF–GP1b-α receptor interaction. This is modelled in our simulations by considering exclusive bonding behaviour, meaning that one monomer can only bind one receptor in the colloid surface. This implies that in order for the polymer to bind another colloid it must remain attached to at least one colloid for enough time such that on average another colloid collides with it and a link between both is formed through the polymer. Thus, in terms of the time scales introduced above, when τ 2 > τ 1 , we expect to see clusters form. It is interesting to note that the collision time and the rotation time scale are of the same order. This effect actually helps strengthen the formation of the aggregate because each polymer can wrap around and form multiple bonds with each of the colloids on the same time scale in which colloids are colliding. Furthermore, the ‘capture area’ per colloid, defined as the area fraction of a colloid that can bind another colloid, increases dramatically from this wrapping mechanism. Note that this effect is completely absent in the case in which the surface of the colloids would be sticky by itself, as in this case there is no enhancement of the bond strength from the rotational component of the flow. In fact, shear flow tends to break such aggregates as intuitively expected. This is shown explicitly in Supplementary Fig. S2 , where we show how shear flow only breaks pure colloidal aggregates. It is important to mention, however, that at low shear rates flow drives the formation of such colloid–colloid aggregates because the collision time in the absence of flow is limited by diffusion, which is extremely slow for these large colloids/platelets. Polymer–colloid aggregates inspired by the process of blood plugging appear to be a new class of self-assembled materials that display universal properties, as shown by our simulations. To finalize our discussion, however, it is of interest to compare the simulation results with the experimental results. In particular, we would like to extract microscopic properties from this comparison, such as the binding energy and force between polymer and colloids. We observe experimentally that the aggregation process occurs around ≈4,000s −1 . As mentioned previously, the characteristic timescale for vWF τ ≈10 −4 s, which implies that we expect the binding energy to be in between the lowest binding energy we have studied here of 4 k B T and the intermediate energy of 5 k B T. Along the reaction coordinate, the distance between the binding minima and the top of the barrier for the GPIbα–vWF A1 pair has been experimentally measured to be ~2 nm [28] . This gives a bond breakup force of the order of ~10 pN that is in excellent agreement with experiments [28] , [29] . In summary, we have presented experimental and simulation results inspired by blood clotting at large flow rates that show unambiguously that polymers and colloids containing complementary associating groups can be induced to form composites with tunable morphologies determined by the strength of the flow. Notice that this system does not aggregate below a critical shear rate or in quiescent conditions. The exact critical shear rate can be controlled by the intramolecular forces in the biopolymer as shown in the simulations where coiled polymers (ideal chains) lead to aggregation much more readily than collapsed globules. The conformation of the polymers can be regulated by chemical or physical means, as for example changing the pH or temperature. We believe that such control of the conformation of vWF may be important in biology to regulate the formation of plugs only at regions of lesion, without having multiple clot formation elsewhere that can lead to blood-clotting disorders. We have also shown that flow-induced polymer–colloid composite formation is a universal process that can be described by a single parameter that compares the timescale-associated colloid rotation and collision to the timescale for unbinding of the ligand–receptor pairs. The polymer–colloid composites reported here can potentially be used to create novel composites with tunable mechanical, chemical or optical properties. For example, one can tune the degree of branching (measured as the number of bound polymers per colloid) of the composite purely by flow as shown in Supplementary Fig. S6 . In this respect, one can also think of designing clusters with prescribed yielding behaviour that would respond to flow in a very precise way and change their chemical characteristics by exposing hidden chemical groups [30] . In terms of optical properties, it could be possible to use these random aggregates as pigments [31] . In conclusion, we believe that the formation of these aggregates represents a new paradigm in non-equilibrium self-assembly in flow with exciting applications and implications in a wide range of fields. Simulation technique Polymers and colloids are simulated with standard simulating techniques under the framework of fluctuating LB hydrodynamics [25] , [26] in three-dimensional grids with resolutions N x × N y × N z =64 × 32 × 32. Periodic boundary conditions are used in both the x and y directions, and a solid bounce-back boundary condition [26] is used in the z direction. For simplicity, we set the lattice spacing Δx and LB time step Δt equal to unity. We use N c =32 colloids with radius r c =2.5, the volume fraction of the colloids is φ c ≈3%. Each polymer consists of N =40 monomers with radius a =0.25. The total number of polymers is N p =128, and the volume fraction of the polymers is φ p ≈0.5%. To control the solvent property of the polymers, we add a Lennard–Jones potential between each monomers with strength u . It has been shown that u =0.41 and 2.08 k B T are suitable choices for simulating polymers in the Θ and bad solvent [19] , [20] . The monomers interact with the binding sites on the colloid surfaces (where each colloid has N b =64 binding sites on the surface) through the Bell model [21] . In the Bell model, the binding and unbinding probability for a reaction pair are P B =exp(− E B / k B T ) and P UB =exp(−( E UB −fr 0 )/ k B T ), where E B and E UB are the binding and unbinding energy barriers, f the average force loaded on the bond and r 0 the characteristic bond length that we set r 0 =0.01 a for all the simulations. In order to have a good averaging of the bond force f , and for the unbinding monomers to have enough time to diffuse away from its bound partner [23] , [24] , in the simulations the binding and unbinding attempts are performed every 100 LB time steps ( τ 0 =100). Effectively, the binding and unbinding time scales for a bond are τ B ≈ τ 0 exp( E B / k B T ) and τ UB ≈ τ 0 exp( E UB / k B T ) [23] , [24] . Other parameters for the fluid are the density ρ =1, the kinematic viscosity ν =1/6 and the temperature k B T =5 × 10 −5 . The characteristic monomer diffusion time is thus τ =6 πηa 3 / k B T ≈10 3 , where η = νρ is the dynamic viscosity of the fluid. Experimental methods For analysis of vWF–platelet and vWF–colloid aggregates, we used freshly taken whole-blood samples. Natrium–citrat was added to ensure anticoagulation and prevention of platelet activation during flow experiments. For vWF–platelet mixture, plasma was replaced with a solution of fluorescent-labelled recombinant vWF (Baxter, Vienna, Austria) in PBS in order to bring the vWF concentration in whole blood to 50 μg ml −1 . For vWF–colloid mixture, plasma was replaced as described above and platelets were substituted with passively coated glass spheres in a concentration of 200,000 per μl of blood. These borosilicate glass spheres (Duke Scientific, Palo Alto, USA) with a diameter of 2 μm were biofunctionalized by linkage of Polyclonal Rabbit Anti-Human vWF (DakoCytomation, Glostrup, Denmark). The antibody linkage to glass beads succeeds by a multistep process by linkage of the vWF antibody to the base-treated microspheres via mal-PEG-NHS (alpha-Maleinimido-omega-carboxy succinimidyl ester polyethylene glycol, Iris Biotech GmbH, Marktredwitz, Germany). This complex PEGlycation process is thoroughly described elsewhere [32] . As negative control, samples of platelets and colloids, respectively, were prepared as described above without addition of recombinant vWF. In a further experimental setting, vWF–platelet mixture was supplemented with 50 μg ml −1 monoclonal inhibitor of human GPIb-α (ImmunoTools, Friesoythe, Germany) to completely block the interaction of GPIb-α receptor on the surface of platelets with the A1 domain of vWF. For distinct shear rate applications, we used air-pressure-driven microfluidic channels (BioFlux, San Francisco, CA, USA) mimicking human microvasulature, coated with recombinant vWF with a concentration of 50 μg ml −1 . Biofunctionalization of the channels with vWF was done by filling the channels with the vWF solution and incubation of the channels for 3 h at 37 °C in a moisture-rich environment. Study of the vWF–platelet/vWF–colloid mixture adhesion to the biofunctionalized channel succeeds by application of a Zeiss Axio Observer Z.1 (Carl Zeiss AG, Oberkochen, Germany) capable of performing fluorescence and reflection interference contrast microscopy (RICM). RICM was used to study the interference pattern of polarized incoming light being reflected at an object in order to reconstruct the height profile of the object at an interface. Briefly, the interference of the object beam and the reference beams results in an image with information on the height profile of the sample. For reduction of scattered light, we utilize antiflex technique in which the incident light passes a linear polarizer. Consequently, RICM technique assures confirmation of colloids coming in direct contact with the observed surface in a high spatial resolution. Image acquisition and analysis was performed using AxioVision software (Carl Zeiss AG). How to cite this article: Chen, H. et al . Blood-clotting-inspired reversible polymer-colloid composite assembly in flow. Nat. Commun. 4:1333 doi: 10.1038/ncomms2326 (2013).